Proteomic screen reveals Fbw7 as a modulator of the NF-κB pathway Fbw7 is a ubiquitin-ligase that targets several oncoproteins for proteolysis, but the full range of Fbw7 substrates is not known. Here we show that by performing quantitative proteomics combined with degron motif searches, we effectively screened for a more complete set of Fbw7 targets. We identify 89 putative Fbw7 substrates, including several disease-associated proteins. The transcription factor NF-κB2 (p100/p52) is one of the candidate Fbw7 substrates. We show that Fbw7 interacts with p100 via a conserved degron and that it promotes degradation of p100 in a GSK3β phosphorylation-dependent manner. Fbw7 inactivation increases p100 levels, which in the presence of NF-κB pathway stimuli, leads to increased p52 levels and activity. Accordingly, the apoptotic threshold can be increased by loss of Fbw7 in a p100-dependent manner. In conclusion, Fbw7-mediated destruction of p100 is a regulatory component restricting the response to NF-κB2 pathway stimulation. Fbw7 is the substrate recognition component of the Skp1-Cul1-F-box (SCF) ubiquitin-ligase SCF Fbw7 (ref. 1 ). SCF Fbw7 acts as a central node by targeting several oncogenic regulators of proliferation, growth and apoptosis for proteasomal degradation. These include cyclin E [2] , c-Myc [3] , Notch [4] and Mcl1 (ref. 5 ). Deletion of the FBW7 gene results in developmental defects, embryonic lethality [3] , [6] and genetic instability [7] and inactivation of FBW7 by loss of expression or mutation [8] has been firmly associated with tumour development [1] , [9] . However, a detailed understanding of the full set of Fbw7 substrates, how regulation of its various substrates is coordinated, and how Fbw7 inactivation causes disease is still lacking. Fbw7 binds to substrates through interaction between its WD40 repeats [10] and a degron motif in the substrate. This binding commonly requires phosphorylation of the substrate's degron on the serine (S) or threonine (T) residues by Glycogen synthase kinase 3 (GSK3) [11] . The occurrence of multiple degrons in Fbw7 substrates has been suggested to increase their affinity to Fbw7 or make the interaction more likely to occur [10] , [12] , [13] . NF-κB2 belongs to the NF-κB family of transcription factors that regulate the expression of several hundred genes and thereby the response to various stimuli such as cytokines and stress [14] . The NF-κB pathway is implicated in numerous diseases, in particular cancer and immune disorders, and is extensively explored as a therapeutic target. The NF-κB protein family also includes RelA, RelB, c-Rel and NF-κB1 (p105/p50). These proteins regulate transcription by complex formation, commonly RelA:p50 dimers, referred to as the canonical and RelB:p52 dimers referred to as the non-canonical NF-κB pathway [15] . The p100 protein has a dual role in transcription as the precursor of p52 and an I-κB-like inhibitor [16] . Although initially described as distinct pathways, the canonical and the non-canonical NF-κB pathways are now shown to share components and to be regulated in an integrated manner [17] . To screen for a more complete set of Fbw7 substrates, we performed quantitative proteomics using FBW7 knockout (KO) cells, combined with bioinformatic analysis of degron motifs. We identified 89 putative Fbw7 substrates, including several disease-associated fundamental regulators of cell fate. Here we found NF-κB2 as one of the candidate Fbw7 substrates and show that Fbw7 ubiquitylates p100 and promotes its degradation in a GSK3β-dependent manner. Fbw7 inactivation causes elevated p100 levels, which in the presence of NF-κB pathway stimuli leads to increased p52 activity. We also show that the apoptotic threshold can be increased by loss of Fbw7 in a p100-dependent manner. This study provides insights into how inactivation of Fbw7 and constitutive activation of the NF-κB pathway might contribute to tumorigenesis. Quantitative proteomics Several of the previously identified SCF Fbw7 targets have elevated protein levels in the human colorectal cancer cell-line HCT116 with homozygous deletion of the FBW7 gene, compared with its wild-type (WT) counterpart. To systematically identify candidate SCF Fbw7 substrates, we performed quantitative proteomics comparing HCT116 FBW7 WT and FBW7 KO cells. A schematic representation of the experimental design is outlined in Fig. 1a . Cytosolic and nuclear/organelle-enriched fractions from biological replicates of each cell type were subjected to isobaric labelling, using Tandem mass tags (TMT) [18] and the relative protein levels were determined by mass spectrometry (MS). More than 7,000 proteins were identified and quantified using peptide HiRIEF (high-resolution isoelectric focussing) LC-MS/MS (liquid chromatography tandem mass spectrometry) ( Supplementary Table S1 ). Approximately 1,700 unique proteins were found at significantly different levels in KO cells, including the known Fbw7 substrates Cyclin E, mTOR, KLF5, c-Myc and TGIF [2] , [19] , [20] , [21] , which, as expected, were upregulated in KO cells. Using Ingenuity pathway analysis, several pathways associated with the differentially expressed proteins were identified, including those related to known Fbw7 substrates such as c-Myc and mTOR ( Supplementary Table S2 ). 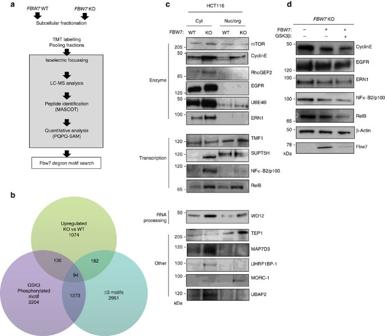Figure 1: Identification of SCFFbw7substrates. (a) Screen design and proteomic workflow for global identification of candidate Fbw7 targets. Subcellular fractionation of HCT116FBW7WT and KO cells into cytosolic (Cyt) and nuclear-/organellar-(Nuc/org) enriched fractions was followed by TMT labelling, sample pooling and peptide fractionation by HiRIEF. Analysis of quantitative data by PQPQ46-SAM identified upregulated proteins. (b) Venn diagram showing the total number and overlap of (1) the proteins found by quantitative proteomics to be upregulated in KO cells (2) proteins with ≥3 Fbw7 degron motifs (RKS/TPRKXS/T/E/D) and (3) proteins with motifs predicted to be phosphorylated by GSK3. (c) Validation of quantitative MS-data. WB analysis comparing endogenous protein levels in the different fractions from WT and KO cells. Equal protein amount from each cell type were analysed. (d)FBW7KO cells were transiently transfected with Fbw7 and GSK-3β as indicated for 24 h. Whole cell extracts were analysed by WB. Figure 1: Identification of SCF Fbw7 substrates. ( a ) Screen design and proteomic workflow for global identification of candidate Fbw7 targets. Subcellular fractionation of HCT116 FBW7 WT and KO cells into cytosolic (Cyt) and nuclear-/organellar-(Nuc/org) enriched fractions was followed by TMT labelling, sample pooling and peptide fractionation by HiRIEF. Analysis of quantitative data by PQPQ [46] -SAM identified upregulated proteins. ( b ) Venn diagram showing the total number and overlap of (1) the proteins found by quantitative proteomics to be upregulated in KO cells (2) proteins with ≥3 Fbw7 degron motifs ( RK S/TP RK XS/T/E/D) and (3) proteins with motifs predicted to be phosphorylated by GSK3. ( c ) Validation of quantitative MS-data. WB analysis comparing endogenous protein levels in the different fractions from WT and KO cells. Equal protein amount from each cell type were analysed. ( d ) FBW7 KO cells were transiently transfected with Fbw7 and GSK-3β as indicated for 24 h. Whole cell extracts were analysed by WB. Full size image Fbw7 degron motif analysis To filter out non-substrates from the pool of upregulated proteins, we combined the proteomic data with searches for proteins with the Fbw7 degron motif. Based on earlier studies of the cyclin E degrons [10] and analysis of the hydrophobicity and isoelectric point of the amino acids surrounding characterized degrons ( Supplementary Fig. S1 ), searches were made for the sequence RK S/TP RK XS/T/E/D, where X is any amino acid and RK is any amino acid except arginine (R) or lysine (K) [11] . Distribution of this motif and variations was analysed proteome-wide and in the different protein pools identified in the proteomics experiment. Proteins with the motif were significantly enriched in the pool of upregulated and depleted in the pool of downregulated nuclear/organelle proteins. The cytoplasmic pools showed no significant enrichment for proteins with Fbw7 motifs ( Supplementary Fig. S2a ). Most of the known SCF Fbw7 substrates contain multiple degron motifs ( Supplementary Table S3 ). Interestingly, the relative size of the fraction of proteins with a given minimum number of motifs grows as that number increases, for known substrates compared with the proteome, suggesting that proteins with multiple motifs are more likely to be substrates ( Supplementary Fig. S2b ). We therefore examined the occurrence of multiple Fbw7 degron motifs as well. To account for phosphorylation of degrons, we used Netphos [22] to predict phosphorylation sites in the motifs. Based on these analyses, 89 putative substrates were selected ( Supplementary Data 1 ). The selection process is further explained in Supplementary Fig. S2c and summarized in Fig. 1b . All established Fbw7 substrates determined to be significantly changed by the proteomics analysis passed the selection process supporting the reliability of this strategy for discovery of Fbw7 substrates ( Supplementary Data 1 ). The list of candidate substrates includes oncoproteins such as EGFR and RhoGEF-2. In addition, proteins with functions not previously associated with SCF Fbw7 substrates, like phosphatases and structural proteins were found ( Supplementary Fig. S3 ). A total of 16 proteins were analysed by western blot (WB) to confirm the MS-based quantification data showing higher endogenous protein levels in FBW7 KO cells ( Fig. 1c ). Moreover, five candidates were tested by analysing their levels on ectopic expression of Fbw7 or Fbw7 together with active GSK3β, in the KO cells. As would be expected for substrates, restoring Fbw7 expression decreased the steady-state levels of these proteins ( Fig. 1d ). NF-κB2 ubiquitylation and levels are regulated by Fbw7 One of the more interesting novel SCF Fbw7 substrates was the Nuclear Factor of κB2 (NF-κB2), also named p100/p52. RelB was also identified as a potential Fbw7 substrate in the proteomic screen and as shown in Fig. 1c , both p100 and RelB were elevated in HCT116 FBW7 KO cells compared with the WT cells. Analysis of p100 and RelB protein half-life following inhibition of protein synthesis by cycloheximide treatment showed reduced turnover rate of both proteins in the KO cells ( Fig. 2a and b ). 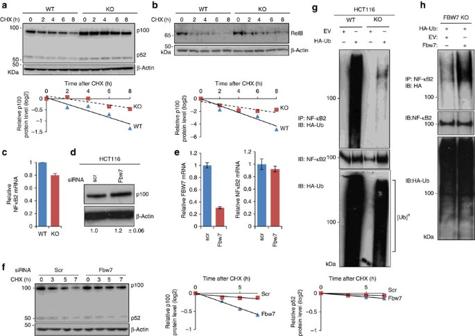Figure 2: NF-κB2 ubiquitylation and levels are regulated by Fbw7. (a) p100 turnover rate is prolonged inFBW7KO HCT116 cells. p100 protein half-life was analysed following treatment with cycloheximide. p100 band intensity was normalized to β−actin and then normalized to t=0 controls. p100 half-life in WT=6.7 h (R2=0.87) and in KO=14.7 h (R2=0.78) (b) RelB turnover rate is prolonged inFBW7KO HCT116 cells. RelB protein half-life was measured as in (a). WT=1.9 h (R2=0.91) and in KO=4.6 h (R2=0.71) (c) Total RNA was prepared from WT and KO cells andNF-κB2mRNA expression was analysed by qRT–PCR. The results are shown as means. Error bars indicate s.d. (n=3). (d) p100 protein levels increase on Fbw7 silencing. HCT116FBW7WT cells were transfected with the scrambled (scr) orFBW7siRNA for 48 h. Endogenous p100 protein was analysed by WB. ±indicated s.d. (n=3). (e) qRT–PCR ofFBW7andNF-κB2mRNA levels from siRNA transfected cells in (d), n=3, error bars indicate s.d. (f) Fbw7 knockdown stabilizes p100 protein. HEK293 cells were transfected with the indicated siRNAs for 48 h and NIK for 24 h and treated with cycloheximide. p100 and p52 half-lives were analysed. The graphs to the right show quantification of the protein bands in the blot. p100 half-life control=12 h (R2=0.99) and Fbw7=58 h (R2=0.72). Degradation of p52 was marginal under these conditions and time frames. (g) Fbw7 ubiquitylates endogenous p100.FBW7WT and KO cells were transfected with HA-ubiquitin. NF-κB2 was immunoprecipitated from whole-cell extracts and NF-κB2 ubiquitylation was analysed by WB using HA antibodies (see also methods). (h) Ubiquitylation of endogenous p100 is restored by ectopic Fbw7 expression.FBW7KO cells were transiently transfected with FBW7. Ubiquitination assay was performed as described in (g). Figure 2: NF-κB2 ubiquitylation and levels are regulated by Fbw7. ( a ) p100 turnover rate is prolonged in FBW7 KO HCT116 cells. p100 protein half-life was analysed following treatment with cycloheximide. p100 band intensity was normalized to β−actin and then normalized to t=0 controls. p100 half-life in WT=6.7 h (R 2 =0.87) and in KO=14.7 h (R 2 =0.78) ( b ) RelB turnover rate is prolonged in FBW7 KO HCT116 cells. RelB protein half-life was measured as in ( a ). WT=1.9 h (R 2 =0.91) and in KO=4.6 h (R 2 =0.71) ( c ) Total RNA was prepared from WT and KO cells and NF-κB2 mRNA expression was analysed by qRT–PCR. The results are shown as means. Error bars indicate s.d. ( n =3). ( d ) p100 protein levels increase on Fbw7 silencing. HCT116 FBW7 WT cells were transfected with the scrambled (scr) or FBW7 siRNA for 48 h. Endogenous p100 protein was analysed by WB. ±indicated s.d. ( n =3). ( e ) qRT–PCR of FBW7 and NF-κB2 mRNA levels from siRNA transfected cells in ( d ), n=3, error bars indicate s.d. ( f ) Fbw7 knockdown stabilizes p100 protein. HEK293 cells were transfected with the indicated siRNAs for 48 h and NIK for 24 h and treated with cycloheximide. p100 and p52 half-lives were analysed. The graphs to the right show quantification of the protein bands in the blot. p100 half-life control=12 h (R 2 =0.99) and Fbw7=58 h (R 2 =0.72). Degradation of p52 was marginal under these conditions and time frames. ( g ) Fbw7 ubiquitylates endogenous p100. FBW7 WT and KO cells were transfected with HA-ubiquitin. NF-κB2 was immunoprecipitated from whole-cell extracts and NF-κB2 ubiquitylation was analysed by WB using HA antibodies (see also methods). ( h ) Ubiquitylation of endogenous p100 is restored by ectopic Fbw7 expression. FBW7 KO cells were transiently transfected with FBW7. Ubiquitination assay was performed as described in ( g ). Full size image In this study, we focus on p100 and its potential regulation by Fbw7. Real-time quantitative (qRT) PCR analysis showed a small decrease in p100 mRNA expression in the KO cells, further indicating that higher protein levels are not caused by higher mRNA transcription ( Fig. 2c ). Silencing Fbw7 in WT cells by small interfering RNA (siRNA) confirmed increased p100 protein, but not mRNA levels ( Fig. 2d-e ). We examined the turnover rate of p100 and p52 in Fbw7-silenced HEK293 cells. As shown in Fig. 2f, the half-life of p100 was prolonged in Fbw7-depleted cells. The very low levels of the basally processed p52 protein in these unstimulated cells were essentially unchanged. The levels of the other NF-κB family proteins that were also examined in HCT116 FBW7 WT and KO cells by WB analysis were unaffected ( Supplementary Fig. S4 ). To directly test whether p100 is a ubiquitylation target of Fbw7, we performed in-vivo ubiquitylation assay. HCT116 FBW7 WT and Fbw7 KO cells were transfected with hemagglutinin (HA)-tagged ubiquitin. Immunoprecipitation (IP) of endogenous p100, followed by WB analysis for HA-ubiquitin, showed that poly-ubiquitylation of NF-κB2/p100 was inefficient in KO cells ( Fig. 2g ). Accordingly, NF-κB2 poly-ubiquitylation could be restored by transient Fbw7 expression in the KO cells ( Fig. 2h ). Fbw7 interacts with NF-κB2 through a conserved degron Next, we examined the binding of NF-κB2 to Fbw7 using co-immunoprecipitation analysis. HEK293 cells were transfected with either full-length or F-box deleted (ΔF) Fbw7. Fbw7ΔF can bind to substrates, but not to the SCF core ligase and, therefore, has dominant negative properties [2] . Both WT and ΔF Fbw7 co-purified with immunoprecipitated endogenous NF-κB2/p100 ( Fig. 3a ). Similarly, reciprocal immunoprecipitations showed that NF-κB2 co-purified with GST-tagged Fbw7 ( Fig. 3b ). To map the region in NF-κB2/p100 required for interaction with Fbw7, we used a series of carboxy-terminally truncated NF-κB2 mutants ( Fig. 3c ). Cells were co-transfected with GST-Fbw7ΔF and the indicated NF-κB2 deletion constructs. The 1–859 and 1–735 mutants both bound to Fbw7, but a larger deletion extending to amino acid 665, did not. This indicates that the integrity of the region 665–735 is essential for efficient interaction with Fbw7. The 1–665 mutant lacks a highly conserved Fbw7 degron motif at amino acid 705–711( Fig. 3d ). Accordingly, no interaction between Fbw7 and the 1–445 deletion, corresponding to p52, could be detected ( Fig. 3e ). We also tested the effect of ectopic Fbw7ΔF expression on the steady-state levels of the different NF-κB2 deletion mutants. As anticipated, the levels of the 1–859 and 1–735, but not the 1–665 mutant increased on expression of Fbw7ΔF ( Fig. 3f ). 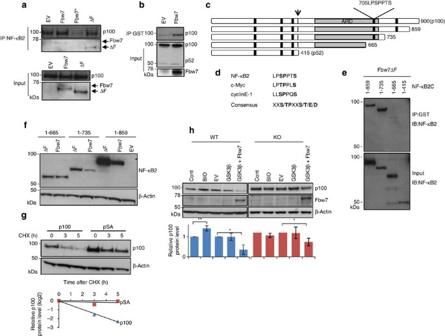Figure 3: Fbw7 interacts with NF-κB2 through a conserved phospho-degron. (a) NF-κB2 binds Fbw7. HEK293 cells were transfected with FLAG-tagged Fbw7 or Fbw7ΔF. Cells were treated with MG132 for 3 h before cell lysis. p100 was immunopurified with anti-NF-κB2 antibodies and Fbw7 binding was analysed by WB using anti-FLAG antibody. * indicates control reaction with beads only. (b) HEK cells were transfected with p100 empty GST vector (EV) or GST-tagged Fbw7. Binding of NF-κB2/p100 protein was analysed following GST-pull-down. (c) Schematic representation of the full-length and different C-terminal NF-κB2 deletions. The arrow indicates the p52 cleavage site. ARD, Ankryn repeat domain. Black boxes indicate putative Fbw7 degron motifs. The motif most similar to known degrons is localized at amino acids 705–711. (d) Comparison of amino acid sequence of the NF-κB2 motif with defined degrons in cyclin E1 and c-Myc. (e) Fbw7 interacts with the NF-κB2 C-terminus. Cells were co-transfected with GST-tagged Fbw7ΔF and the NF-κB2 constructs as indicated. Fbw7 was pulled down with GST-beads followed by WB with anti-NF-κB2 antibody. (f) HEK293 cells were co-transfected with the indicated plasmids and NF-κB2 protein level was analysed by WB. (g) p100 protein with mutated degron motif is stable. Half-life of the WT p100 and the pSA-mutant (serines 707 and 711 replaced by alanines) were compared by CHX-chase analysis in HEK293 cells. The graph shows quantification of the p100 band in the blot on a log2 scale as compared to t=0. (h) GSK-3β induces p100 and RelB degradation by Fbw7. HCT116FBW7WT and KO cells were treated with the GSK3β inhibitor (BIO) or transfected with empty vector, GSK3β or GSK3β and Fbw7 as indicated. Lower panel shows quantified relative p100 protein levels. Error bars indicate s.d. One samplet-tests were used to determine statistical significance (n=3 for WT andn=4 for KO). *P<0.05; **P<0.01 and ***P<0.001. Figure 3: Fbw7 interacts with NF-κB2 through a conserved phospho-degron. ( a ) NF-κB2 binds Fbw7. HEK293 cells were transfected with FLAG-tagged Fbw7 or Fbw7ΔF. Cells were treated with MG132 for 3 h before cell lysis. p100 was immunopurified with anti-NF-κB2 antibodies and Fbw7 binding was analysed by WB using anti-FLAG antibody. * indicates control reaction with beads only. ( b ) HEK cells were transfected with p100 empty GST vector (EV) or GST-tagged Fbw7. Binding of NF-κB2/p100 protein was analysed following GST-pull-down. ( c ) Schematic representation of the full-length and different C-terminal NF-κB2 deletions. The arrow indicates the p52 cleavage site. ARD, Ankryn repeat domain. Black boxes indicate putative Fbw7 degron motifs. The motif most similar to known degrons is localized at amino acids 705–711. ( d ) Comparison of amino acid sequence of the NF-κB2 motif with defined degrons in cyclin E1 and c-Myc. ( e ) Fbw7 interacts with the NF-κB2 C-terminus. Cells were co-transfected with GST-tagged Fbw7ΔF and the NF-κB2 constructs as indicated. Fbw7 was pulled down with GST-beads followed by WB with anti-NF-κB2 antibody. ( f ) HEK293 cells were co-transfected with the indicated plasmids and NF-κB2 protein level was analysed by WB. ( g ) p100 protein with mutated degron motif is stable. Half-life of the WT p100 and the pSA-mutant (serines 707 and 711 replaced by alanines) were compared by CHX-chase analysis in HEK293 cells. The graph shows quantification of the p100 band in the blot on a log2 scale as compared to t=0. ( h ) GSK-3β induces p100 and RelB degradation by Fbw7. HCT116 FBW7 WT and KO cells were treated with the GSK3β inhibitor (BIO) or transfected with empty vector, GSK3β or GSK3β and Fbw7 as indicated. Lower panel shows quantified relative p100 protein levels. Error bars indicate s.d. One sample t -tests were used to determine statistical significance ( n =3 for WT and n =4 for KO). * P <0.05; ** P <0.01 and *** P <0.001. Full size image As Fbw7 substrate recognition and subsequent degradation depends on prior phosphorylation of the degron, we examined the turnover rate of an NF-κB2/p100 mutant in which the serines in the predicted GSK3 phosphorylation sites, S707 and S711, were replaced by alanines (p100-SA). As shown in Fig. 3g , the p100-SA mutant had a markedly increased half-life as compared with WT p100. To address how phosphorylation by GSK3β affects Fbw7-mediated regulation of p100, we compared p100 levels in FBW7 WT and KO cells following GSK3β inhibition or activation. In WT cells, treatment with the pharmacological GSK3β-inhibitor BIO increased the levels of p100, whereas ectopic expression of active GSK3β together with Fbw7 reduced p100 levels efficiently ( Fig. 3h ). In contrast, no increase in p100 levels after GSK3β inhibition was detected in the KO cells, indicating that Fbw7-dependent modulation of p100 takes place following phosphorylation by GSK3β. Fbw7 modulates p100/p52 levels and activity To examine whether Fbw7-mediated ubiquitylation of p100 also affects its partial degradation to p52, p100 processing was induced by expression of the NF-κB inducing kinase (NIK), a direct activator of the non-canonical NF-κB pathway [23] . p52 production was not perturbed in response to NIK stimulation in Fbw7-silenced HEK cells, indicating that in contrast to the SCF ubiquitin-ligase βTrCP, ubiquitination by Fbw7 is not required for p100 processing ( Fig. 4a ). Interestingly, p52 protein levels were higher in Fbw7-depleted cells following stimulation by NIK. Similarly, we observed higher p52 levels on NIK stimulation of cells expressing the dominant-negative Fbw7ΔF in all replicates, whereas cells expressing WT Fbw7 showed a concomitant decrease of both p100 and p52 proteins ( Fig. 4b ). In addition, on stimulation of the non-canonical pathway by CD40 Ligand (CD40L) in MDA-231 cells ectopically expressing Fbw7, p52 levels were lower, suggesting that the steady-state level of the precursor p100 is reduced by Fbw7 and is rate-limiting for inducible p52 production in response to stimulation of the CD40 receptor as well ( Fig. 4c ). 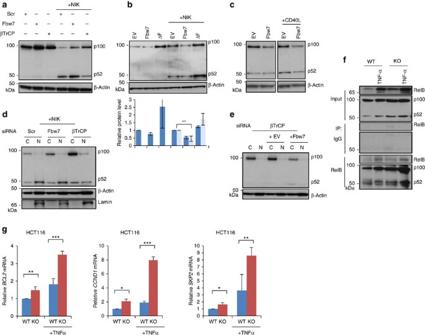Figure 4: Fbw7 modulates p100/p52 levels and activity. (a) Fbw7 knockdown increases p52 protein levels. HEK293 cells were transfected with control (scr), Fbw7 or βTrCP siRNA oligos followed by transient transfection of p100 with or without NIK for 24 h. Whole-cell extracts were analysed. (b) Fbw7 alters p100 and p52 levels. HEK293 cells were co-transfected with p100 and Fbw7 or Fbw7ΔF, with or without NIK and analysed by WB. Lower panel shows quantified protein levels, for p100 (dark bars) and p52 (light bars). Error bars indicate s.d. (n=3, Fbw7+NIKn=5). (c) Fbw7 reduces p52 levels on CD40 stimulation. MDA-231 cells were transfected with control (EV) or Fbw7 plasmid. 24 h post-transfections cells were stimulated by soluble recombinant CD40 overnight and analysed by WB. (d) HEK293 cells were transfected with control (scr), Fbw7 or βTrCP siRNAs followed by transient transfection of p100 and NIK for 24 h. p100 levels in the cytosolic and nuclear extracts were analysed. (e) HEK293 cells were transfected with βTrCP siRNA oligos followed by transient transfection of control (EV) or Fbw7 for 24 h. p100 levels in the cytosolic and nuclear extracts were analysed. (f) p52:RelB complexes are more abundant inFBW7KO cells. HCT116FBW7WT and KO cells were treated with 10 ng ml−1TNF-α for 24 h before lysis. 200 μg of protein was used to immunoprecipitate RelB. (g) Increased mRNA expression of NF-κB2 targets inFBW7-deficient cells.FBW7WT and KO cells were treated or not with 10 ng ml−1TNF-α for 24 h before total RNA extraction. qPCR was performed for the indicated genes. Actin was used as a normalizing gene and all levels were compared with untreated WT. Graph depicts the mean and s.d. of a minimum of three independent experiments. Statistical significance was tested using ANOVA. *P<0.05; **P<0.01 and ***P<0.001. Figure 4: Fbw7 modulates p100/p52 levels and activity. ( a ) Fbw7 knockdown increases p52 protein levels. HEK293 cells were transfected with control (scr), Fbw7 or βTrCP siRNA oligos followed by transient transfection of p100 with or without NIK for 24 h. Whole-cell extracts were analysed. ( b ) Fbw7 alters p100 and p52 levels. HEK293 cells were co-transfected with p100 and Fbw7 or Fbw7ΔF, with or without NIK and analysed by WB. Lower panel shows quantified protein levels, for p100 (dark bars) and p52 (light bars). Error bars indicate s.d. ( n =3, Fbw7+NIK n =5). ( c ) Fbw7 reduces p52 levels on CD40 stimulation. MDA-231 cells were transfected with control (EV) or Fbw7 plasmid. 24 h post-transfections cells were stimulated by soluble recombinant CD40 overnight and analysed by WB. ( d ) HEK293 cells were transfected with control (scr), Fbw7 or βTrCP siRNAs followed by transient transfection of p100 and NIK for 24 h. p100 levels in the cytosolic and nuclear extracts were analysed. ( e ) HEK293 cells were transfected with βTrCP siRNA oligos followed by transient transfection of control (EV) or Fbw7 for 24 h. p100 levels in the cytosolic and nuclear extracts were analysed. ( f ) p52:RelB complexes are more abundant in FBW7 KO cells. HCT116 FBW7 WT and KO cells were treated with 10 ng ml −1 TNF-α for 24 h before lysis. 200 μg of protein was used to immunoprecipitate RelB. ( g ) Increased mRNA expression of NF-κB2 targets in FBW7 -deficient cells. FBW7 WT and KO cells were treated or not with 10 ng ml −1 TNF-α for 24 h before total RNA extraction. qPCR was performed for the indicated genes. Actin was used as a normalizing gene and all levels were compared with untreated WT. Graph depicts the mean and s.d. of a minimum of three independent experiments. Statistical significance was tested using ANOVA. * P <0.05; ** P <0.01 and *** P <0.001. Full size image Knockdown of either Fbw7 or βTrCP caused accumulation of p100 in unstimulated cells. Following NIK-stimulation of βTrCP-silenced cells, p100 remains predominantly unprocessed in the cytoplasm but in Fbw7-silenced cells, p100 is processed and p52 translocated to the nucleus ( Fig. 4d ). Notably, ectopic expression of Fbw7 in cells accumulating p100 as a result of processing block by βTrCP knockdown leads to a decrease in the levels of unprocessed, cytoplasmic p100 ( Fig. 4e ). We also investigated the production of p52 on stimulation of cells with TNF-α, which is primarily an activator of the canonical pathway. Unlike NIK that directly induces processing of p100 to p52, TNF-α stimulation contributes indirectly to increased p52 levels, likely through inducing p100 transcription, as p100 is a transcriptional target of the canonical NF-κB pathway [24] , [25] . TNF-α treatment further enhanced p52 levels in KO compared with WT cells. IP of the endogenous p52 with anti-RelB antibodies showed that p52:RelB complexes are more abundant in basal and in TNF-α stimulated FBW7 -KO cells ( Fig. 4f ). This is interesting as complex formation between p52 and RelB is a prerequisite for transcriptional activation of a subset of p52 targets [15] . To investigate the effect of Fbw7-mediated control of p100 on the non-canonical NF-κB pathway activity, we performed transcription assays. Consistent with the increased abundance of p52:RelB complexes in stimulated FBW7 KO cells, expression of p52-specific targets Cyclin D1, Bcl2 and Skp2 was higher in these cells, as shown by qPCR analysis of relative messenger RNA levels ( Fig. 4g ). In support of the inhibitory role of p100 on NF-κB activity [26] , we observed that in unstimulated HCT FBW7 KO cells with higher p100 levels, basal NF-κB activity was lower when compared with WT cells ( Fig. 5a ). Also, overexpression of p100 or the p100SA mutant suppressed κB-TATA reporter activity in unstimulated HEK and HCT cells ( Fig. 5b ). However, on stimulation of cells by NIK, κB-TATA promoter activity was recovered. NIK- and prolonged TNF-α-stimulated HCT cells showed a higher fold-induction of the relative κB-TATA activity in FBW7 KO compared with WT cells ( Fig. 5c ). This indicates that induction of processing in cells with elevated p100 levels can lead to a greater response to stimulation. Gene-specific luciferase assay in U2OS cells, which have constitutively active p100 processing [15] , demonstrated that expression of Fbw7ΔF increases cyclin D1 promoter activity ( Fig. 5d ). Similarly, stimulated Fbw7ΔF-expressing HEK cells showed an enhanced κB-TATA activity ( Fig. 5e ). Moreover, we detected increased protein levels of Cyclin D1, Bcl-2 and Skp2 following TNF-α stimulation in FBW7 KO cells ( Fig. 5f ). 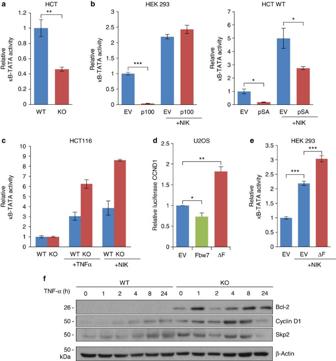Figure 5: Regulation of NF-κB activity by Fbw7 with or without stimuli. (a) Basal NF-κB activity is lower in HCT116FBW7KO compared with WT cells. WT and KO cells were transfected with the kB-luciferase reporter. Relative luciferase activity was measured. Results are shown as means. Error bars indicate s.d. (n=3). (b) p100 overexpression represses kB-luciferase activity in the absence of stimulation. HEK293 or HCTFBW7WT cells were transfected with the kB-luciferase reporter and empty vector (EV), p100, pSA and NIK as indicated. Results are shown as means. Error bars indicate s.d. (n=3). The p100/EV ratios of fold induction were 29 (s.d.=5) in HEK and 2.9 (s.d.=0.75) in HCT cells. (c)FBW7WT and KO cells were transfected with the κB-Luciferase reporter with NIK or treated with 5 ng ml−1TNF-α (24 h). Luciferase activity was analysed and normalized to untreated cells for each cell type. Error bars show s.d. (n=3). (d) U2OS cells were transfected with EV, Fbw7 or Fbw7ΔF as indicated. All cells were also transfected with the cyclin D1 promoter-specific luciferase reporter. Results are shown as means. Error bars indicate s.d. (n=3). (e) Response to the NF-κB pathway stimulation is enhanced in Fbw7ΔF expressing cells. HEK293 cells were transfected with the κB-Luciferase reporter and NIK, Fbw7 and Fbw7ΔF as indicated for 48 h. Luciferase activity was measured. The results were shown as means. Error bars are s.d. (n=3). (f) Protein levels of NF-κB2 targets are higher inFBW7KO cells. WB analysis of NF-κB2 targets in HCTFBW7WT and KO cells. Cells were treated with 10 ng ml−1TNF-α for the indicated times. Statistical significance was tested using ANOVA in (d) and unpaired, two-tailedt-tests elsewhere. *P<0.05; **P<0.01 and ***P<0.001. Figure 5: Regulation of NF-κB activity by Fbw7 with or without stimuli. ( a ) Basal NF-κB activity is lower in HCT116 FBW7 KO compared with WT cells. WT and KO cells were transfected with the kB-luciferase reporter. Relative luciferase activity was measured. Results are shown as means. Error bars indicate s.d. ( n =3). ( b ) p100 overexpression represses kB-luciferase activity in the absence of stimulation. HEK293 or HCT FBW7 WT cells were transfected with the kB-luciferase reporter and empty vector (EV), p100, pSA and NIK as indicated. Results are shown as means. Error bars indicate s.d. ( n =3). The p100/EV ratios of fold induction were 29 (s.d.=5) in HEK and 2.9 (s.d.=0.75) in HCT cells. ( c ) FBW7 WT and KO cells were transfected with the κB-Luciferase reporter with NIK or treated with 5 ng ml −1 TNF-α (24 h). Luciferase activity was analysed and normalized to untreated cells for each cell type. Error bars show s.d. ( n =3). ( d ) U2OS cells were transfected with EV, Fbw7 or Fbw7ΔF as indicated. All cells were also transfected with the cyclin D1 promoter-specific luciferase reporter. Results are shown as means. Error bars indicate s.d. ( n =3). ( e ) Response to the NF-κB pathway stimulation is enhanced in Fbw7ΔF expressing cells. HEK293 cells were transfected with the κB-Luciferase reporter and NIK, Fbw7 and Fbw7ΔF as indicated for 48 h. Luciferase activity was measured. The results were shown as means. Error bars are s.d. ( n =3). ( f ) Protein levels of NF-κB2 targets are higher in FBW7 KO cells. WB analysis of NF-κB2 targets in HCT FBW7 WT and KO cells. Cells were treated with 10 ng ml −1 TNF-α for the indicated times. Statistical significance was tested using ANOVA in ( d ) and unpaired, two-tailed t -tests elsewhere. * P <0.05; ** P <0.01 and *** P <0.001. Full size image Elevated p100 on Fbw7 loss is pro-survival when processed To assess the consequence of Fbw7-mediated control of p100 on cell fate, we performed viability and apoptosis analysis. Deregulation of the NF-κB2 pathway has been shown to be essential for cell survival by controlling the expression of anti-apoptotic genes, for example, in lymphomas [27] . However, unprocessed p100 has also been reported to induce apoptosis through non-transcriptional as well as transcriptional processes [28] , [29] . Cell survival in response to treatment with the anticancer drugs Daunorubicin, Doxorubicin and Etoposide, known to be affected by the NF-κB pathway, was analysed [30] , [31] . We show that in U2OS cells, that have constitutive p100 processing, knockdown of Fbw7 decreased sensitivity to Daunorubicin and Etoposide treatment and knockdown of p100 reversed the pro-survival effect resulting from Fbw7 loss ( Fig. 6a-c ). Consistently, ectopic expression of the p100SA mutant, resistant to degradation by Fbw7, reduced apoptosis in response to Doxorubicin in NIK-stimulated HEK293 cells ( Fig. 6d ). Together, these data support a pro-survival effect of p100 deregulation as a result of Fbw7 loss in cells with activated p100 processing. 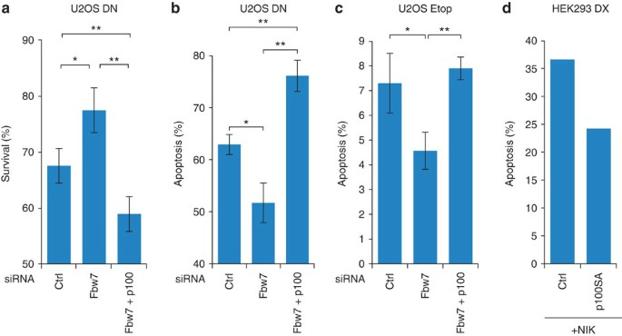Figure 6: Elevated p100 as a result of Fbw7 loss increases survival when processed. (a) U2OS cells were transfected with the control (scrambled), Fbw7 or/and p100 siRNA as indicated. 48-h post-silencing cells were treated with 1 μM Daunorubicin (DN) for 48 h and cell survival was assayed by crystal violet staining. (b) Cells were treated with 1 μM DN for 48 h and apoptosis was monitored by Annexin V staining. (c) Cells were transfected as inaand treated with 10 μM Etoposide (Etop) for 24 h. Apoptosis was monitored by Annexin V staining. (d) HEK293 cells were transiently transfected with the mutant p100 (p100SA) and NIK and treated with 1 μM Doxorubicin (DX) for 29 h and subjected to Annexin V staining. Welch'st-test was used to determine statistical significance in all panels (n=3). Error bars indicate s.d. *P<0.05; **P<0.01 and ***P<0.001. Figure 6: Elevated p100 as a result of Fbw7 loss increases survival when processed. ( a ) U2OS cells were transfected with the control (scrambled), Fbw7 or/and p100 siRNA as indicated. 48-h post-silencing cells were treated with 1 μM Daunorubicin (DN) for 48 h and cell survival was assayed by crystal violet staining. ( b ) Cells were treated with 1 μM DN for 48 h and apoptosis was monitored by Annexin V staining. ( c ) Cells were transfected as in a and treated with 10 μM Etoposide (Etop) for 24 h. Apoptosis was monitored by Annexin V staining. ( d ) HEK293 cells were transiently transfected with the mutant p100 (p100SA) and NIK and treated with 1 μM Doxorubicin (DX) for 29 h and subjected to Annexin V staining. Welch's t -test was used to determine statistical significance in all panels ( n =3). Error bars indicate s.d. * P <0.05; ** P <0.01 and *** P <0.001. Full size image Consistent with a role for p52 in tumorigenesis, we found elevated protein levels of p100/p52 in several primary paediatric B-cell Acute lymphoblastic leukaemia (B-ALL) ( Supplementary Fig. S5 ). To investigate a potential relationship between Fbw7 and NF-κB2 in B-ALL, we performed correlation analysis for the expression of Fbw7 and specific NF-κB2 target genes in two independent cohorts of 178 and 297 patients. Considering expression as a continuous variable, a highly significant inverse association was found between the expression of Fbw7 and several NF-κB2 target genes, such as Bcl2 and Bcl2L1 ( Supplementary Table S4 ). Quantitative proteomics analysis is a logical choice for E3-ligase target studies. However, high analytical depth is essential for successful identification of target proteins. Here we used HiRIEF LC-MS/MS to quantify over 7,000 proteins. A combination of conservative bioinformatic criteria was then applied to separate primary and downstream effects with minimal loss of information. By this method, we identify NF-κB2 as a novel Fbw7 target. Our data suggests that a pool of p100 is constitutively phosphorylated by GSK3β, ubiquitinated by Fbw7 and degraded independently of stimulation of the NF-κB pathway. Although inhibition of either Fbw7 or βTrCP leads to increased p100 levels, the distribution pattern of p100 and p52 protein is clearly distinct in stimulated cells, under each condition. Stimulation of Fbw7-deficient cells leads to increased p52 levels consistent with the higher expression of p52-specific targets in these cells. Based on our findings, we present a model for how Fbw7 modulates the NF-κB pathway activity in normal and diseased cells ( Fig. 7 ). Normally, p100 is the prevalent form of NF-κB2 and processing to p52 is restricted [16] , but in response to stimulation, p100 processing is transiently triggered in a NIK- and βTrCP-dependent manner [16] , [32] . Our results suggest that the control of p100 levels by Fbw7-mediated ubiquitylation and proteolysis is decisive for the extent of the transcriptional response on stimulation, as Fbw7-deficient cells with elevated p100 levels have increased p52 activity leading to increased cell survival. This is intriguing since inactivation of Fbw7 and/or activation of NF-κB2 (p52) is a frequent event in various tumour types, including haematological malignancies [33] , [34] , [35] . The inverse correlation between expression of Fbw7 and specific NF-κB2 target genes that we found in ALL underscores the link between Fbw7 and NF-κB2 in tumorigenesis. Moreover, considering the interconnected nature of the NF-κB network of transcription regulators [36] , we suggest that control of p100 levels by Fbw7 is likely to be a general modulator of response to stimulation of both the NF-κB pathways. 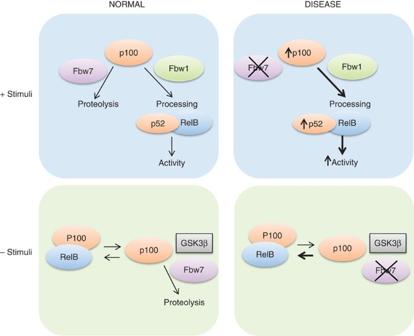Figure 7: Fbw7 modulates the response to NF-κB pathway stimulation through controlling p100 protein levels. In response to specific stimuli p100 is processed to p52 through NIK-mediated phosphorylation. Increase in p100 levels as a result of Fbw7 inactivation leads to elevated p52 production, alterations in p52/NF-κB complex formation and activity on stimulation. In the absence of stimuli, p100 binds to and inhibits various NF-κB complexes. Consequently, Fbw7-mediated regulation of p100 levels controls downstream transcriptional targets of both the canonical (RelA:p50) and the non-canonical (RelB:p52) NF-κB pathways. Figure 7: Fbw7 modulates the response to NF-κB pathway stimulation through controlling p100 protein levels. In response to specific stimuli p100 is processed to p52 through NIK-mediated phosphorylation. Increase in p100 levels as a result of Fbw7 inactivation leads to elevated p52 production, alterations in p52/NF-κB complex formation and activity on stimulation. In the absence of stimuli, p100 binds to and inhibits various NF-κB complexes. Consequently, Fbw7-mediated regulation of p100 levels controls downstream transcriptional targets of both the canonical (RelA:p50) and the non-canonical (RelB:p52) NF-κB pathways. Full size image During the final stages of the preparation of this manuscript, we became aware of another study demonstrating that efficient activation of the non-canonical NF-κB pathways is dependent on the elimination of a nuclear pool of p100 through either degradation by Fbw7 or export to cytoplasm [28] . This study also shows that in multiple myeloma cell lines, accumulation of unprocessed p100 is pro-apoptotic. There is previous evidence for both a pro- and anti-apoptotic role of p100 under distinct conditions [27] , [29] . While unprocessed p100 has been shown to be primarily pro-apoptotic, we show that elevated p100, when processed to p52 is pro-survival. Thus, the outcome of Fbw7-mediated modulation of p100 levels on cell survival is different under distinct modes of NF-κB pathway activation. Unlike in multiple myeloma cell lines, in many other cancer types Fbw7 is inactivated, consistent with a pro-survival role for deregulated p100 as a result of Fbw7 deficiency. In the present study we provide a novel technique for systematic discovery of SCF Fbw7 ubiquitin-ligase substrates that could readily be adapted for other ubiquitin-ligases. The identified candidates are proteins with greater functional diversity than previously anticipated for Fbw7 substrates, and further studies of these targets would provide a more complete understanding of Fbw7 function and how its deregulation causes disease. In cancer, the NF-κB signalling is often dysregulated and constitutively activated [37] . Through study of p100 regulation by Fbw7, we provide insights into how inactivation of Fbw7 together with constitutive activation of the NF-κB pathway might contribute to tumorigenesis. Note added in proof: Similar findings have been reported while this work was under consideration (Fukushima et al . Cell Rep . 1 , 434–443, 2012. SCFFbw7 modulates the NFκB signaling pathway by targeting NFκB2 for ubiquitination and destruction). Cell culture and transfections Human embryonic kidney HEK293 and human osteosarcoma U2OS cell lines were cultured in DMEM (Invitrogen). Human colorectal carcinoma cell lines HCT116 FBW7 +/+ (WT) and HCT116 FBW7 −/− (KO) were cultured in McCoy's medium (Invitrogen). All cells were supplemented with 10% fetal calf serum at 37 °C in 5% CO 2 . Cells were treated with the proteasome inhibitor MG132 (Sigma) at 40 μM, Cycloheximide (Sigma) at 100 μg ml −1 , TNF-α (Prepotech) at 5–10 ng ml −1 , GSK3β inhibitor Bromoindirubin (Sigma) at 5 μM for 3 h. Soluble hexa-meric CD40 ligand (ENZO Life Science) was used 0.4 μg ml −1 , over night. FBW7 plasmids and transfections were performed as previously described [8] , [39] using TransIT-LT1 (Mirus) reagent or GeneJuice Transfection Reagent (Novagen). Transfection of siRNA oligonucleotides was performed with HiPerfect transfection reagent (Qiagen) for 48 h. Fbw7 siRNA has been described previously [39] . βTrCP siRNA was a kind gift from Dr. Guardavaccaro. Full-length and C-terminal deletion NF-κB2 deletion constructs and NIK vectors were described previously [23] . GSK3β plasmid was a kind gift from Dr. Theresa Vincent. The double-point mutant of p100, where serine 707 and serine 711 was replaced by alanines (p100-SA), was generated using the Quickchange kit, according to the manufacturer's instructions (Stratagene). Immunoprecipitation and immunoblotting Nuclear- and cytosolic-enriched fractions were prepared as described previously [14] . Whole-cell lysate preparation, immunoprecipitation and immunoblotting have been described previously [39] , [40] . Antibodies: anti-NF-κB2 (Santa Cruz) (2 μg ml −1 ) and (Sigma) (1 μg ml −1 ), anti cyclin E (Santa Cruz) 0.4 μg ml −1 , anti-HA (Santa Cruz) 1 μg ml −1 , anti-β-actin (Sigma) (1:5,000), anti-FLAG M2 (Sigma) (1:1,000). Antibodies to Bcl-2 (1:1,000), Cyclin D1 (1:1,000), Skp2 (1:1,000) were obtained from Cell Signaling Technology. Antibodies to RhoGEF2 (2 μg ml −1 ), EGFR (0.2 μg ml −1 ), UBE4B (0.05 μg ml −1 ), ERN1 (2 μg ml −1 ), TMF1 (0.5 μg ml −1 ), SUPT5 H (0.4 μg ml −1 ), WD12 (0.2 μg ml −1 ), TEP1 (0.1 μg ml −1 ), MAP7D3 (1 μg ml −1 ), UHRF1BP1 (2 μg ml −1 ), MORC-1 (0.4 μg ml −1 ), UBAP2 (0.2 μg ml −1 ) were from Human Protein Atlas antibodies. In-vivo ubiquitination assays were performed essentially as described previously [41] . Briefly, HCT116 (WT and KO) cells were transfected with a plasmid expressing HA-ubiquitin for 24 h and treated with MG132 (50 μM) for 6 h before collectinging and extraction in 1% SDS and 10 mM N -ethylmaleimide (Sigma). Protein extracts were sonicated, diluted ten times in RIPA buffer followed by immunoprecipitation of equal amounts of total NF-κB2 protein using anti-NF-κB2 antibodies. Pathway analysis The proteins identified by MS were studied for their biological function and pathways. Basic information about the proteins was retrieved from UniProt/SwissProt database (release 2011-06). These proteins were also analysed using ingenuity pathway analysis (IPA version 9, release date 2011-03-12). Reporter assays and mRNA expression analysis Luciferase reporter assays were carried out using the Dual-Luciferase Reporter Assay System (Promega), according to the manufacturer's instructions. κB-responsive gene-specific reporters from the Cyclin D promoter [40] and the Bcl-2 promoter (a kind gift from Professor Neil Perkins) were used. κB- TATA luciferase reporter has been described previously [25] . Renilla was used for normalization. Luciferase reporter experiments were repeated three times. Total RNA was extracted using TRIzol reagent (Invitrogen) and reverse-transcribed into complementary DNA by using Superscript reverse transcriptase (Invitrogen) followed by quantitative RT–PCR (qRT–PCR) analysis, as described previously [42] . Gene expression levels were analysed on an ABI 7300 Real-Time PCR System (SDS software version 1.3.1) and normalized, based on GAPDH mRNA expression. Primer sequences are indicated in Supplementary Table S5 . For Bcl-2, Quantitate SYBR-validated primers were used (Qiagen). Gene-specific mRNA expression levels were determined by Affymetrix U133 plus 2.0 GeneChips, as previously described in ref. 43 . Relations between continuous variables were investigated by means of the Spearman's rank correlation coefficient test. A P -value of <0.05 was considered to indicate statistical significance. Sample preparation for Proteomics Protein extracts of the two subcellular fractions were precipitated by acetone. The resulting pellets were dissolved in 1% SDS, with subsequent stepwise dilutions to 0.1%SDS. After estimation of the total protein amount (Bio-Rad DC), to each aliquot containing 40 μg of total protein, TEAB pH 8.5 was added (25 mM final conc.). After reduction of cysteines by dithiothreitol and carbamidomethylation by IAA, samples were digested by trypsin (sequencing grade modified, Promega). The resulting peptide mixtures were labelled with TMT (Thermo Scientific) and then pooled into the subcellular sets. After sample cleanup by solid phase extraction (SPE strata-X-C, Phenomenex), the two pools were subjected to peptide IEF-IPG (isoelectric focussing by immobilized pH gradient) in the pI range 3.7–4.9 (ref. 44 ). From each pool, 72 IEF peptide fractions were eluted by liquid handling robotics (GE Healthcare prototype) into a 96-well plate (V-bottom, Corning product #3894), which was then dried in a SpeedVac. LC-ESI-LTQ-Orbitrap MS/MS For each run, the auto sampler (HPLC 1200 system, Agilent Technologies) dispensed 8 μl of solvent A to the well in the 96 V plate, mixed for 10 min, and proceeded to inject 3 μl into a C18 guard desalting column (Agilent) before a 15-cm long C18 picofrit column (100 μm internal diameter, 5 μm bead size, Nikkyo Technos, Tokyo, Japan) installed on to the nano-electrospray ionization source. Solvent A was 97% water, 3% acetonitrile, 0.1% formic acid; and solvent B was 5% water, 95% acetonitrile, 0.1% formic acid. At a constant flow of 0.4 μl min −1 , the curved gradient went from 2%B up to 40%B in 45 min, followed by a steep increase to 100%B in 5 min. Online LC-MS was performed using a hybrid LTQ-Orbitrap Velos mass spectrometer (Thermo Scientific). Precursors were isolated with a 2 m/z window. We enabled 'preview mode' for Fourier transform mass spectrometry (FTMS) master scans, which proceeded at 30,000 resolution (profile mode). Data-dependent MS/MS (centroid mode) followed in two stages: first, the top five ions from the master scan were selected for collision-induced dissociation (CID, at 35% energy) with ion trap mass spectrometry (ITMS) detection; and after, the same five ions underwent higher energy collision dissociation (HCD, at 45% energy) with detection in the orbitrap (FTMS). The entire duty cycle lasted ~3.5 s. Dynamic exclusion was used with 90-s duration. Proteomics data analysis The MS raw files were searched with a target-decoy approach using Mascot 2.3. (Matrix Science) followed by Percolator 1.17 (build date 2010-10-30) [44] under the software platform Proteome Discoverer 1.3.0.339 (Thermo) against the human SwissProt Fasta protein database ( http://www.uniprot.org [45] , release 2011-07). We used a precursor ion mass tolerance of 10 p.p.m., and product ion mass tolerances of 0.02 Da for HCD-FTMS and 0.8 Da for CID-ITMS. The algorithm considered tryptic peptides with at the most one missed cleavage, oxidation (M) as variable modification, and carbamidomethylation (C) and TMT6plex (K, N-term) as fixed modifications. Generated protein and PSM (peptide spectrum match) lists had a 1% false discovery rate (peptide level) cut off. Proteins identified by a single peptide are supplied together with their respective PSMs in Supplementary Data 2 and 3 . TMT reporter ion raw intensities from PSMs corresponding to unique peptides (that is, peptides whose sequence match a unique protein) were subjected to the program PQPQ [46] using a correlation P -value of 0.4. The curated quantitative cross-channel ratios for each protein were logged (base 2) and subsequently analysed with SAM (significance analysis of microarrays [46] , response type: two-class unpaired). Lists of up- and down-regulated proteins were thus obtained with a cutoff at SAM q -value 2%. The proteomics data have been deposited in the PRIDE partner repository Proteome Exchange ( http://proteomecentral.proteomexchange.org ) with the dataset identifier PXD000005. Raw and search result files are available via ftp at ftp://ftp.pride.ebi.ac.uk/2012/06/PXD000005/ or alternatively via SweStore at https://webdav.swegrid.se/snic/bils/ki_scilife/pub/nc.arabi_etal_2012.pdf Bioinformatics and motif analysis The canonical human subset of Swiss-Prot was downloaded from http://www.uniprot.org [45] on 28 October 2011 and searched for non-overlapping matches to regular expressions corresponding to the motif definitions. Netphos 3.1b [22] was used to predict phosphorylation sites for GSK3 and other kinases in the human protein set. The protein lists produced by the proteomics data analysis were mapped onto the canonical subset of proteins by truncation of the protein identifier for non-canonical isoforms and each protein was assigned the smallest q -value as determined by SAM [47] of any variety detected by PQPQ [45] . SciPy and NumPy ( http://www.scipy.org ) were used for statistical calculations and plots produced by Matplotlib ( http://www.matplotlib.sf.net ). Quantification of immunoblot band intensities was performed using Fiji/ImageJ. mRNA expression correlation analysis Relations between continuous variables were investigated by means of the bivariate, two-tailed Spearman's rank correlation coefficient test. A P -value of <0.05 was considered to indicate statistical significance. PASW statistics 17 statistical package was used. Accession codes : The proteomics data have been deposited in the PRIDE partner repository Proteome Exchange ( http://proteomecentral.proteomexchange.org ) under the dataset identifier PXD000005 . Raw and search result files are available via ftp at ftp://ftp.pride.ebi.ac.uk/2012/06/PXD000005/ or alternatively via SweStore at https://webdav.swegrid.se/snic/bils/ki_scilife/pub/nc.arabi_etal_2012.pdf . How to cite this article: Arabi, A. et al . Proteomic screen reveals Fbw7 as a modulator of the NF-κB pathway. Nat. Commun. 3:976 doi: 10.1038/ncomms1975 (2012).